All-thiol-stabilized Ag44and Au12Ag32nanoparticles with single-crystal structures Noble metal nanoparticles stabilized by organic ligands are important for applications in assembly, site-specific bioconjugate labelling and sensing, drug delivery and medical therapy, molecular recognition and molecular electronics, and catalysis. Here we report crystal structures and theoretical analysis of three Ag 44 (SR) 30 and three Au 12 Ag 32 (SR) 30 intermetallic nanoclusters stabilized with fluorinated arylthiols (SR=SPhF, SPhF 2 or SPhCF 3 ). The nanocluster forms a Keplerate solid of concentric icosahedral and dodecahedral atom shells, protected by six Ag 2 (SR) 5 units. Positive counterions in the crystal indicate a high negative charge of 4 − per nanoparticle, and density functional theory calculations explain the stability as an 18-electron superatom shell closure in the metal core. Highly featured optical absorption spectra in the ultraviolet–visible region are analysed using time-dependent density functional perturbation theory. This work forms a basis for further understanding, engineering and controlling of stability as well as electronic and optical properties of these novel nanomaterials. Noble metal nanoparticles stabilized by organic ligand layer are the subject of an increasing number of studies owing to their applications in assembly, bio-labelling and sensing, drug delivery and medical therapy, molecular recognition and molecular electronics, and catalysis. [1] , [2] , [3] , [4] , [5] , [6] , [7] , [8] , [9] , [10] Size, composition and surface structure are important factors determining the physical, chemical and biological properties of monolayer-protected noble metal nanoparticles. [4] , [11] , [12] To achieve chemical fine-tuning, understanding of their structures at the molecular level is crucial. [13] , [14] , [15] Thiol-stabilized Au nanoclusters represent an important class of noble metal nanoparticles whose molecular structures have been characterized by X-ray single-crystal diffractions [15] , [16] , [17] , [18] , [19] and successfully adopted to precisely tailor their electronic and surface properties. [20] , [21] However, in contrast to thiol-stabilized Au nanoclusters, no crystal structure determination has been reported on all-thiol-protected silver nanoparticles, although Ag or Au/Ag nanoclusters with uniform size and even with precise number of atoms have been widely achieved. [22] , [23] , [24] , [25] , [26] , [27] , [28] , [29] , [30] , [31] , [32] , [33] Here we report on the first successful crystal structure determination and theoretical analysis of six all-thiol-protected silver and silver-gold intermetallic nanoparticles, namely three Ag 44 (SR) 30 and three Au 12 Ag 32 (SR) 30 nanoclusters stabilized with fluorinated arylthiols (SR=SPhF, SPhF 2 or SPhCF 3 ). The metal core forms a Keplerate solid of concentric icosahedral and dodecahedral atom shells, protected by six Ag 2 (SR) 5 units in octahedral geometry. The crystal unit cell includes positive counterions indicating a high negative charge of 4 − per nanocluster, and density functional theory (DFT) calculations confirm the expected electronic structure with an 18-electron superatom shell closure in the metal core. The nanoparticles display highly featured optical absorption spectra in the ultraviolet–visible region, and the theoretical analysis of the transitions reveals an important role played by the electron-rich ligand layer. Our results form a basis for further understanding, engineering and controlling of stability as well as electronic and optical properties of these interesting building blocks of novel nanomaterials. Synthesis A typical synthesis of [M 12 Ag 32 (SR) 30 ] 4− clusters involved the chemical reduction of metal precursors (that is, AgBF 4 and ClAuPPh 3 ) by an aqueous NaBH 4 in the presence of fluorinated arylthiol and PPh 4 Br in a mixed solvent of dichloromethane and methanol at 0 °C in an ice bath (see Methods for details). The crystallization of [M 12 Ag 32 (SR) 30 ] 4− clusters was performed by layering hexane into the CH 2 Cl 2 solutions of clusters at 4 °C. Slow recrystallization led to the formation of high-quality millimeter-sized single crystals ( Supplementary Fig. S1a ) for single-crystal analysis. 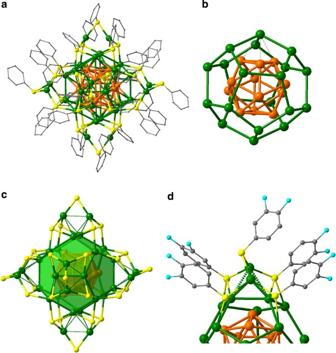Figure 1: Representative crystal structure of the [M12Ag32(SR)30]4−(M=Ag, Au) cluster. (a) The overall structure of the [M12Ag32(SPhF2)30]4−cluster. All hydrogen and fluorine atoms are omitted for clarity. (b) The two-shell M12@Ag20core of the cluster. (c) The arrangement of six [Ag2(SPhF2)5] motif units on the surface of the cluster. (d) The structure of the surface [Ag2(SPhF2)5] motif. Colour legend: orange sphere, M (Ag/Au); green sphere, Ag; yellow sphere, S; cyan sphere, F; grey stick/sphere, C. Six different single crystals containing all-thiol-protected silver and silver-gold intermetallic clusters were successfully obtained depending on the fluorinated arylthiol used and also whether the Au precursor was introduced ( Table 1 and Supplementary Tables S1–S6 ). The obtained crystals are readily dissolved in organic solvents, such as CH 2 Cl 2 and DMF, to give transparent brown solutions ( Supplementary Fig. S1b ). It is noteworthy that one-batch synthesis of [M 12 Ag 32 (SR) 30 ] 4− clusters on a scale of tens of grams has been achieved by scaling up the reaction ( Supplementary Fig. S2 ). Table 1 A summary of crystallographic data for selected synthesized clusters with various surface thiolates*. Full size table Atomic structure As revealed by single-crystal analysis, all of the six crystals containing [M 12 Ag 32 (SR) 30 ] 4− (M=Ag, Au) clusters co-crystallized with PPh 4 + . Each cluster consists of a Keplerate two-shell M 12 @Ag 20 core protected by six Ag 2 (SR) 5 units on its surface ( Fig. 1a ). [34] , [35] The core of [M 12 Ag 32 (SR) 30 ] 4− clusters can be depicted as two concentric icosahedral and dodecahedral metal shells. The first shell is a hollow icosahedral cage of M 12 . The 20 M 3 faces of the icosahedral M 12 cage are fully face-capped by Ag atoms to form a two-shell M 12 @Ag 20 cage in a nearly perfect I h point symmetry ( Fig. 1b ). The M–M distances in the first M 12 shell are averaged at 2.780 and 2.829 Å, respectively, for the case of [Au 12 Ag 32 (SPhF 2 ) 30 ] 4− and [Ag 44 (SPhF 2 ) 30 ] 4− . 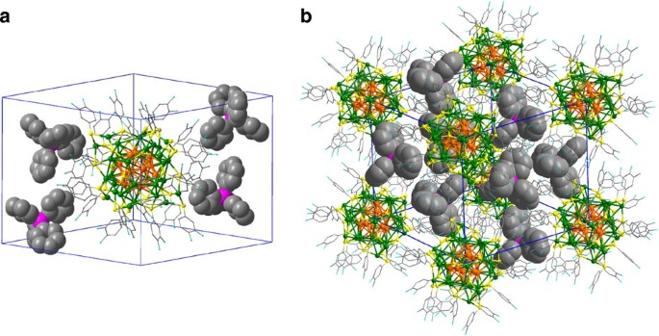Figure 2: The representative packing structures of [M12Ag32(SR)30]4−clusters with PPh4+counterions. (a) Compound 2, (PPh4)4[Au12Ag32(SC6H3F2)30]; (b) Compound 6, (PPh4)4[Au12Ag32(SC6H4CF3)30]. The PPh4+counterions are highlighted in the space-filling style for better visualization. Colour legend: orange sphere, Au; green sphere, Ag; yellow sphere, S; pink sphere, P; grey sphere, C; cyan sphere, F. All hydrogen atoms are omitted for clarity. As shown in Table 2 , the average M–M bond lengths in the first M 12 shell in all [M 12 Ag 32 (SR) 30 ] 4− clusters are slightly shorter than the M–M distance (2.884 Å for Au and 2.889 Å for Ag) in bulk face-centered cubic Au/Ag. The M–Ag distances between the M 12 core and the Ag 20 shell are also slightly smaller than those in bulk face-centered cubic Au/Ag, suggesting the strong bonding between the M 12 shell and Ag 20 shell. Each M 12 @Ag 20 Keplerate cage is capped by six Ag 2 (SR) 5 units to form the [M 12 Ag 32 (SR) 30 ] 4− cluster ( Fig. 1c ). Each of the six Ag 2 (SR) 5 units is connected to an edge of the Ag 20 pentagonal dodecahedron through Ag–SR interactions. The six edges connected to Ag 2 (SR) 5 units have an octahedral symmetry implicit in the Ag 20 pentagonal dodecahedron. As shown in Fig. 1d , the two Ag atoms on the edge of the dodecahedron and the two Ag atoms in each Ag 2 (SR) 5 unit are positioned in a tetrahedral configuration on the surface of the Ag 20 pentagonal dodecahedron. Figure 1: Representative crystal structure of the [M 12 Ag 32 (SR) 30 ] 4− (M=Ag, Au) cluster. ( a ) The overall structure of the [M 12 Ag 32 (SPhF 2 ) 30 ] 4− cluster. All hydrogen and fluorine atoms are omitted for clarity. ( b ) The two-shell M 12 @Ag 20 core of the cluster. ( c ) The arrangement of six [Ag 2 (SPhF 2 ) 5 ] motif units on the surface of the cluster. ( d ) The structure of the surface [Ag 2 (SPhF 2 ) 5 ] motif. Colour legend: orange sphere, M (Ag/Au); green sphere, Ag; yellow sphere, S; cyan sphere, F; grey stick/sphere, C. Full size image Table 2 A summary of important average bond length data for selected synthesized [M 12 Ag 32 (SR) 30 ] 4− clusters. Full size table One of the novel features of [M 12 Ag 32 (SR) 30 ] 4− clusters reported here is the presence of hollow M 12 cage at its core, which is distinguishing from all reported thiolated Au/Ag nanoclusters whose structures have been crystallographically determined. The hollow M 12 cage in [Au 12 Ag 32 (SPhF 2 ) 30 ] 4− and [Ag 44 (SPhF 2 ) 30 ] 4− has an internal diameter (from vertex to vertex) of 5.288 and 5.381 Å, respectively, which represents the possibly smallest Au/Ag cage that can exist (for radial analysis of the atomic structure, see Supplementary Fig. S3 ). Both experimental and theoretical studies have suggested that the pure icosahedral Au 12 is unstable and has to be stabilized by endohedral encapsulation of transition metal atoms. In [M 12 Ag 32 (SR) 30 ] 4− , the hollow M 12 cage is stabilized by being encapsulated in the Ag 20 cage. The presence of the hollow Au 12 cage leads to a very unusual bonding situation that there are no 12-coordinated metal atoms in [M 12 Ag 32 (SR) 30 ] 4− clusters. Each M atom in the first shell of the cluster is coordinated to five M atoms in the same shell and five Ag atoms from the second shell. As a result, the maximum coordination number of metal atoms in the cluster is 10. Besides the presence of hollow M 12 cage and the core-shell distribution of Au and Ag atoms, another striking structural feature in [M 12 Ag 32 (SR) 30 ] 4− is a completely different binding geometry of surface thiolates as compared with the well-known RS(M-SR-) x , ( x =1, 2) oligomeric unit found in thiolated Au nanoclusters and in self-assembled monolayers of thiolates on Au(111). [13] At the surface of the thiolate-capped Au clusters, Au(I) cations are linearly coordinated to two thiolate ligands that are also bound to two core Au atoms ( Supplementary Fig. S4 ). In contrast to such a coordination configuration, we find here that the surface layer of the [M 12 Ag 32 (SR) 30 ] 4− cluster consists of six three-dimensional Ag 2 (SR) 5 units in which Ag cations bind to three thiolate ligands in a planar Ag(SR) 3 configuration. The five thiolate ligands in each surface Ag 2 (SR) 5 motif are classified into two groups. Although the four thiolates directly bonded to the Ag atoms on the M 12 @Ag 20 core are threefold coordinated, the one thiolate jointing the outmost Ag(I) cations is twofold coordinated. As shown in Table 2 , the average Ag–S bond lengths in all [M 12 Ag 32 (SR) 30 ] 4− clusters are in the range of 2.54–2.57 Å, which is longer than the Au–S bond lengths revealed in thiolated Au nanoclusters (2.36 Å for Au 102 (p-MBA) 44 and 2.33 Å for [Au 25 (SCH 2 CH 2 Ph) 18 ] − ). Each [M 12 Ag 32 (SR) 30 ] 4− cluster has a charge of 4 − balanced by four tetraphenylphosphonium (PPh 4 + ) counterions. As shown in the crystal packing ( Fig. 2 ), the rigid PPh 4 + counterions are occupying the intercluster space and help to prevent free rotation of clusters. Owing to the rather large size of the clusters, the extra-cluster spaces were calculated to be >36% of the total volume in all the six single crystals containing [M 12 Ag 32 (SR) 30 ] 4− clusters. It is conceivable that the bulky and rigid PPh 4 + counter cations are essential to the successful co-crystallization of the anionic clusters into high-quality single crystals. Figure 2: The representative packing structures of [M 12 Ag 32 (SR) 30 ] 4− clusters with PPh 4 + counterions. ( a ) Compound 2, (PPh 4 ) 4 [Au 12 Ag 32 (SC 6 H 3 F 2 ) 30 ]; ( b ) Compound 6, (PPh 4 ) 4 [Au 12 Ag 32 (SC 6 H 4 CF 3 ) 30 ]. The PPh 4 + counterions are highlighted in the space-filling style for better visualization. Colour legend: orange sphere, Au; green sphere, Ag; yellow sphere, S; pink sphere, P; grey sphere, C; cyan sphere, F. All hydrogen atoms are omitted for clarity. Full size image Electronic structure and optical properties DFT calculations (for technical details see the Methods section) were performed for the full [Au 12 Ag 32 (SR) 30 ] 4− and [Ag 44 (SR) 30 ] 4− particles using 3,4-difluorobenzenethiol SPhF 2 as the ligand. The computationally relaxed structures, starting from the crystal structure, comply well with the experimental crystallographic information, although the metal–metal distances are slightly longer than in the crystal data because of the Perdew–Burke–Ernzerhof (PBE) approximation ( Table 2 ). Analysis of the local charge in metal atoms in the three shells 1 (12 atoms), 2 (20 atoms) and 3 (12 atoms) was performed using the Bader method and the results are shown in Supplementary Table S7 and Supplementary Fig. S5 . The analysis shows clearly that the 12 metal atoms in the innermost shell are neutral (Ag) or slightly negatively charged (Au), whereas the metal atoms in shells 2 and 3, both in contact with the thiolates, are clearly positively charged. Charge analysis also shows a strong polarization of the free end of each ligand attributed to fluorine, which affects mainly the orientation of the ligands on the surface. The ligands tend to maximize dipole–dipole interactions between the fluorine and carbon of the ligands, which lead to slightly displaced pi–pi stacking ( Supplementary Fig. S5 ). Because of the strongly polarized C–F end of the ligands, dipole–dipole electrostatic interactions are expected to have an important contribution to the ligand–ligand interactions. Our estimate for the stabilization energy for one ligand pair is in the range of 0.1–0.2 eV for which the higher value is obtained using dispersion-corrected functionals. Combined with the fact that tens of these weak interactions sum up in the ligand shell, this interaction contributes significantly to the overall stability of the nanocluster. Supplementary Figures S6 and S7 show the analysis of the ground-state electronic structure of [Au 12 Ag 32 (SR) 30 ] 4− and [Ag 44 (SR) 30 ] 4− , respectively. As expected from the superatom electron-counting rules indicating 18-shell electrons, [36] , [37] both clusters show clear symmetries of 1D [10] for the highest occupied molecular orbital (HOMO) manifold and 2S [2] for the lowest unoccupied molecular orbital (LUMO) states. The calculated HOMO-LUMO gaps are 1.00 eV and 0.77 eV for [Au 12 Ag 32 (SR) 30 ] 4− and [Ag 44 (SR) 30 ] 4− , respectively. Further, three observations can be made: (i) the degeneracies of the superatom orbitals 1D (occupied) and 1F (unoccupied) are split by the octahedral ligand field of the protecting Ag 2 (SR) 5 units, (ii) in the case of the [Au 12 Ag 32 (SR) 30 ] 4− , the lower part of the D superatom shell is merged into the band of the upper ligand states and (iii) the 2S shell is energetically very close to the 1F shell. This special destabilization of 2S is due to the caged atomic structure that enforces the radial node of the 2S state between the 1st and 2nd atomic shells in the cage thus increasing the energy of the state. The destabilization of the 2S state and stabilization of the 18-electron configuration by this mechanism has previously been reported from calculations for (Au 16 ) 2− dianion in a tetrahedral cage structure. [38] As shown in Fig. 3 , the experimental ultraviolet–visible spectra of [Ag 44 (SR) 30 ] 4− clusters in solutions exhibit broad multiband optical absorption that is similar to the clusters reported by Stellacci and coworkers [22] The optical gaps for the [Ag 44 (SR) 30 ] 4− clusters are estimated to be 1.2 eV with absorption tailing up to 1,050 nm. The observed gaps are larger than the computed HOMO-LUMO gap mentioned above (1.00 eV), which is attributed to the fact that the HOMO-LUMO transition (superatom 1D→2S) is dipole-forbidden and the lowest-energy optical transitions are HOMO→LUMO+1, as discussed later. The [Ag 44 (SR) 30 ] 4− clusters display six apparent peaks (at 374, 411, 483, 535, 641 and 833 nm) and two shoulder peaks (at 590 and 689 nm). These absorption bands do not vary with the type of surface thiolates, indicating little influence of thiolate ligands on the absorption of the clusters. However, when the first shell of Ag 12 is substituted by Au 12 , the absorption features of the clusters change dramatically. The [Au 12 Ag 32 (SPhF 2 ) 30 ] 4− and [Au 12 Ag 32 (SPhCF 3 ) 30 ] 4− clusters display only two pronounced peaks at 390 and 490 nm, respectively, although three weak shoulder peaks at 576, 620 and 728 nm are still revealed if carefully examined. In comparison, the two major peaks of [Au 12 Ag 32 (SPhF) 30 ] 4− are red-shifted to 403 and 508 nm. The distinct difference of the optical absorption of [Au 12 Ag 32 (SR) 30 ] 4− from [Ag 44 (SR) 30 ] 4− clusters clearly indicates a significant contribution of the core metal atoms on the overall optical properties of [M 12 Ag 32 (SR) 30 ] 4− clusters. Our optical measurements also revealed that both [Ag 44 (SPhF 2 ) 30 ] 4− and [Au 12 Ag 32 (SPhF 2 ) 30 ] 4− clusters can be stable in their solid form at room temperature in air for at least 6 months ( Supplementary Fig. S8 ). 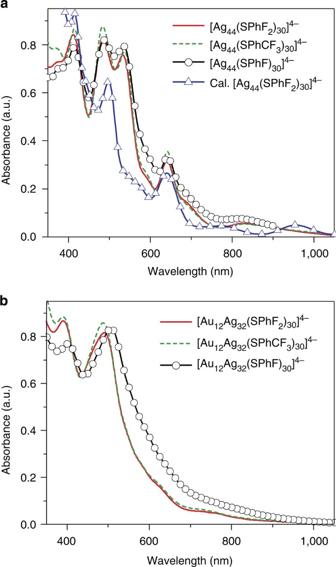Figure 3: Optical properties of [M12Ag32(SR)30]4−clusters. Ultraviolet–visible absorption spectra of (a) [Ag44(SR)30]4−and (b) [Au12Ag32(SR)30]4−clusters with different surface thiolates. Calculated spectrum of [Ag44(SPhF2)30]4−is shown inafor comparison. The dominant features in the theoretical spectrum are analysed inFig. 4andSupplementary Fig. S9. The theoretical spectrum is scaled for comparable intensities with the experimental data in the region of 400–1,000 nm. Figure 3: Optical properties of [M 12 Ag 32 (SR) 30 ] 4− clusters. Ultraviolet–visible absorption spectra of ( a ) [Ag 44 (SR) 30 ] 4− and ( b ) [Au 12 Ag 32 (SR) 30 ] 4− clusters with different surface thiolates. Calculated spectrum of [Ag 44 (SPhF 2 ) 30 ] 4− is shown in a for comparison. The dominant features in the theoretical spectrum are analysed in Fig. 4 and Supplementary Fig. S9 . The theoretical spectrum is scaled for comparable intensities with the experimental data in the region of 400–1,000 nm. Full size image Linear-response time-dependent DFT (TDDFT) calculations were performed for the [Ag 44 (SPhF 2 ) 30 ] 4− cluster and the computed absorption spectrum was compared with the experimental data in Fig. 3 . The theoretical absorption spectrum displays six clear features at 954 nm (1.30 eV), 775 nm (1.60 eV), 642 nm (1.93 eV), 561 nm (2.21 eV), 500 nm (2.48 eV) and 416 nm (2.98 eV) in the spectral range of 400–1,000 nm and allows for assignment of most of the experimentally observed transitions. To decipher the contribution of the states to the dominant peaks, we performed analysis based on time-dependent density functional perturbation theory (for technical details see Methods ) of the calculated spectrum ( Fig. 4 ; Supplementary Figs S9 and S10 ). The two lowest-energy, lowest-intensity transitions (theory values 954 and 775 nm and observed at 833 and 689 nm) are dominantly metal-to-metal superatom 1D→1F type (HOMO→LUMO+1). The calculated peaks are red-shifted by about 0.2 eV. Previous theoretical work on the well-known Au 25 (SR) 18 1− cluster by Aikens et al . [39] has shown that shifts of this magnitude are within the general inaccuracies of the DFT functionals, particularly taking into account the fact that the PBE functional slightly overestimates the metal–metal distances in the M 12 Ag 20 nanoparticle core ( Table 2 ). The clear experimental peak at 641 nm, reproduced also from the theory extremely well (642 nm), has a mixed character of metal-to-metal 1D→1F and ligand-to-1F. The two dominant peaks in the computed spectrum at 416 and 500 nm are solely of the type superatom 1D→ligand and Ag(4d)+ligand→superatom 1F type. The electron-hole densities corresponding to these higher-energy peaks are delocalized over the full particle including the ligand shell, indicating the crucial contribution of the electron-rich ligands in these collective excitations. We note that it has been experimentally shown that the intensities of the peaks around 500 nm are somewhat dependent on the solvent. [40] A deeper understanding of the character of excitations needs further theoretical work beyond the scope of the present paper. 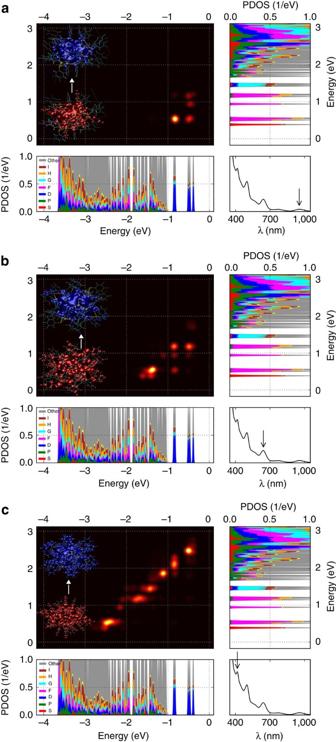Figure 4: Analysis of peaks in the theoretical ultraviolet–visible spectrum of [Ag44(SR)30]4−. Three peaks at (a) 954 nm, (b) 642 nm and (c) 416 nm, all of different characters are shown by the arrows in the bottom right parts of each panel and are analysed from time-dependent density functional perturbation theory TD-DFPT. The horizontal and vertical graphs show electronic density of states for occupied and unoccupied states, respectively, with the colours showing their angular momentum characters (as inSupplementary Figs S6 and S7). The two-dimensional map shows the weights (squares of the absorption coefficient) of the non-interacting KS transitions contributing to the marked peak. In the colour scale, yellow represents the maximum weight. The insets show visualization of the excitation by means of the hole density (density of occupied states involved in the transition). The insets are shown in a larger scale inSupplementary Fig. S10. Figure 4: Analysis of peaks in the theoretical ultraviolet–visible spectrum of [Ag 44 (SR) 30 ] 4− . Three peaks at ( a ) 954 nm, ( b ) 642 nm and ( c ) 416 nm, all of different characters are shown by the arrows in the bottom right parts of each panel and are analysed from time-dependent density functional perturbation theory TD-DFPT. The horizontal and vertical graphs show electronic density of states for occupied and unoccupied states, respectively, with the colours showing their angular momentum characters (as in Supplementary Figs S6 and S7 ). The two-dimensional map shows the weights (squares of the absorption coefficient) of the non-interacting KS transitions contributing to the marked peak. In the colour scale, yellow represents the maximum weight. The insets show visualization of the excitation by means of the hole density (density of occupied states involved in the transition). The insets are shown in a larger scale in Supplementary Fig. S10 . Full size image Our work on the family of six [M 12 Ag 32 (SR) 30 ] 4− nanoclusters highlights several novel features not encountered before in structural studies of thiolate-stabilized noble metal nanoclusters, and implies factors contributing to their stability. First, this study shows an overall robustness of the two-shell Keplerate metal core with respect to varying fluorinated arylthiolates as protecting ligands and allowing the occupation of the innermost 12-atom metal shell either with silver or gold. Second, the novel surface structure of ligands revealed here implies that the medium-sized thiol-stabilized Au nanoclusters doped with other metals could have a surface ligand structure that is distinctly different from those pure thiolate-capped Au nanoclusters (Au 25 , Au 36 , Au 38 and Au 102 ) that have been structurally characterized until now. Third, fluorinated arylthiols are demonstrated here to be effective ligands to stabilize the clusters via enhanced weak interactions in the ligand layer and to cooperate with rigid counterions allowing the growth of high-quality single crystals of macroscopic (mm) size. Such a synthesis and crystallization strategy might also work for structurally yet uncharacterized thiolated Au clusters such as Au 144 . Fourth, a remarkable fulfillment of one of the predictions of superatom shell electron counts of 18 for metal nanoclusters is for the first time realized in these systems. This electronic magic number is related to the cage-like structure of the inner metal core. Fifth, it is demonstrated that alloying gold and silver enhances the thermal stability of the cluster over the all-silver system. Together with the unique electronic and optical properties, the high stability and ease of the scalable synthesis of macroscopic quantities (currently, tens of grams from single batch) of these structurally well-defined silver and gold-silver nanoclusters make it possible to further engineer and optimize their properties for a variety of emerging applications. We expect their widespread use in several laboratories in the near future. Reagents Silver acetate (AgCH 3 COO, 99%), 3,4-difluorothiophenol (C 6 H 4 F 2 S, 98%), 4-fluorothiophenol (C 6 H 5 FS, 96%), 4-(trifluoromethyl)thiophenol (C 7 H 5 F 3 S, 97%), diphenyl-2-pyridylphosphine (C 17 H 14 NP, 97%) and tetraphenylphosphonium bromide (PPh 4 Br, 98%) were purchased from Alfa Aesar Chemical Reagent Co. Ltd. Silver nitrate (AgNO 3 , analytical grade), sodium borohydride (NaBH 4 , 98%), dichloromethane (CH 2 Cl 2 , analytical grade) and methanol (CH 3 OH, analytical grade) were purchased from Sinopharm Chemical Reagent Co. Ltd. (Shanghai, China). The water used in all experiments was ultrapure. All reagents were used as received without further purification. Synthesis of Compound 1 Twenty milligrams of AgNO 3 were dissolved in the mixture solution of dichloromethane and methanol. The solution was cooled to 0 °C in an ice bath, 10 μl 3,4-difluorobenzenethiol, and then 12 mg tetraphenylphosphonium bromide were added. After 20-min stirring, 1 ml NaBH 4 aqueous solution (45 mg ml −1 ) and 50 μl triethylamine were added quickly under vigorous stirring. The reaction was aging for 12 h at 0 °C. The aqueous phase was then removed and the mixture in organic phase was washed several times with water. Black block crystals were crystallized from CH 2 Cl 2 /hexane at 4 °C after 10 days. The yield of compound 1, (PPh 4 ) 4 [Ag 44 (SC 6 H 3 F 2 ) 30 ], was ~70%. Synthesis of Compound 2 Ten milligrams of chloro(diphenyl-2-pyridylphosphine)gold(I) (AuPPh 2 PyCl) and 10 mg AgNO 3 were used instead of 20 mg AgNO 3 in the synthesis of Compound 1. All the other conditions were kept unchanged. The yield of Compound 2, (PPh 4 ) 4 [Au 12 Ag 32 (SC 6 H 3 F 2 ) 30 ], was ~65%. Synthesis of Compounds 3–6 During the synthesis of Compound 1 and Compound 2, 3,4-difluorobenzenethiol was substituted by the same amount of other fluorinated arylthiols (that is, 4-fluorobenzenethiol and 4-trifluoromethylbenzenethiol) while keeping the other conditions the same. The reactions led to the formation of [M 12 Ag 32 (SR) 30 ] 4− clusters stabilized by the corresponding thiols: Compound 3, (PPh 4 ) 4 [Ag 44 (SC 6 H 4 F) 30 ]; Compound 4, (PPh 4 ) 4 [Au 12 Ag 32 (SC 6 H 4 F) 30 ]; Compound 5, (PPh 4 ) 4 [Ag 44 (SC 6 H 4 CF 3 ) 30 ]; and Compound 6, (PPh 4 ) 4 [Au 12 Ag 32 (SC 6 H 4 CF 3 ) 30 ]. Single-crystal analysis of Compounds 1–6 The diffraction data of all single crystals of Compounds 1–6 were collected on an Agilent SuperNova X-Ray single-crystal diffractometer using Cu Kα ( λ =1.54184 Å) and Mo Kα ( λ =0.71069 Å) micro-focus X-ray sources at 100 and 173 K, respectively. The data were processed using CrysAlisPro. The structure was solved and refined using Full-matrix least-squares based on F 2 . More detailed refinement data are provided in Supplementary Tables S1–S6 . The refined electron density maps (2Fo-Fc) and non-biased difference density (Fo-Fc) maps for Compounds 1–6 are also given in Supplementary Figs S11–S16 . Measurements of optical properties Pure crystals of Compounds 1–6 were dissolved in dichloromethane (CH 2 Cl 2 ) for spectrum measurements. Ultraviolet–visible absorption spectra were recorded on a Varian Carry 5000 spectrophotometer. DFT and TDDFT calculations For the computational modelling, we used DFT as implemented in the real-space code-package GPAW (Grid-based projector-augmented wave method). [41] Structure optimization was performed using full ligands as used in the experiment, both PBE and local density approximation functionals, [42] 0.2 Å grid spacing and 0.05 eV/Å convergence criterion for the maximum forces acting on atoms in clusters. The PBE-relaxed structures were used for further analysis. The GPAW set-ups for Au and Ag include scalar-relativistic corrections. Superatom electron state symmetries were analysed by projecting the wave functions to spherical harmonics with respect to the center of mass of the cluster as described in ref. 37 . Optical absorption spectra were calculated for the PBE-relaxed structures using linear-response TDDFT. [43] CCDC Mercury software was used for analysis of weak interaction contacts in the ligand layer. Atomic charges were evaluated by using the Bader method. [44] Ligand–ligand interactions were calculated using two representative ligands of Ag 44 cluster as a separated 3,4-difluorobenzenethiol HSPhF 2 pair. For the ligand–ligand interactions, both PBE and local density approximation functionals were used with GPAW. It was also confirmed that the local charges of the polarized C- and F-atoms were not changed compared with the full cluster model. Ligand–ligand interactions were also checked using Turbomole DFT-code package with dispersive corrections included to both PBE-D and B97-D functionals. Analysis of excitations in the ultraviolet–visible spectra The time-dependent density functional perturbation theory (TD-DFPT) was used to analyse calculated spectral features. [45] , [46] In TD-DFPT, a perturbation expansion of the time-dependent Kohn–Sham (KS) equation is made with respect to the strength of the external electric field, for example, a laser field. We choose a laser field with a single frequency using the frequency of the target spectral feature. The first-order TD-DFPT equation can be written as a set of linear equations in the frequency space. [47] Figure 4 and Supplementary Fig. S9 visualize the elements of the response wavefunction. Each element, that is, a response coefficient, is associated with a KS-occupied state i (hole after the excitation) and an unoccupied state p (electron after the excitation). Traditionally, electron-hole contributions have been analysed for individual transitions pair by pair. However, this is not practical for large systems where tens of interacting transitions—which themselves are composed of tens of non-interacting transitions—can contribute to a single spectral feature. Therefore, we create a ‘transition contribution map’ ( Fig. 4 and Supplementary Fig. S9 ) where the three axes are (1) the eigenvalue of the occupied state, ‘KS hole energy’, (2) the eigenvalue of the unoccupied state, ‘KS electron energy’ and (3) the square of the absorption coefficient, ‘contribution intensity’. Each contribution is broadened by a Gaussian for visualization. Other choices for the first two axes of the transition contribution map are also possible, for example, some spatial projection. Moreover, a transition contribution map can be combined with another analysis method. Here we have combined it with the Y LM (spherical harmonics) analysis showing the superatomic states. Accession codes: The X-ray crystallographic coordinates for structures reported in this article (see Table 1 and Supplementary Data 1–6 ) have been deposited at the Cambridge Crystallographic Data Centre (CCDC) under deposition numbers CCDC 953878 (Compound 1), CCDC 953879 (Compound 2), CCDC 953880 (Compound 3), CCDC 953881 (Compound 4), CCDC 953882 (Compound 5) and CCDC 953883 (Compound 6). These data can be obtained free of charge from the Cambridge Crystallographic Data Centre via http://www.ccdc.cam.ac.uk/data_request/cif . A and B level alerts arising from the checkCIF/PLATON procedure of the cif files are explained by the partial disorder of surface organic ligands on the clusters. How to cite this article: Yang, H. et al . All-thiol-stabilized Ag 44 and Au 12 Ag 32 nanoparticles with single-crystal structures. Nat. Commun. 4:2422 doi: 10.1038/ncomms3422 (2013).